Dicke-type phase transition in a spin-orbit-coupled Bose–Einstein condensate Spin-orbit-coupled Bose–Einstein condensates (BECs) provide a powerful tool to investigate interesting gauge field-related phenomena. Here we study the ground state properties of such a system and show that it can be mapped to the well-known Dicke model in quantum optics, which describes the interactions between an ensemble of atoms and an optical field. A central prediction of the Dicke model is a quantum phase transition between a superradiant phase and a normal phase. We detect this transition in a spin-orbit-coupled BEC by measuring various physical quantities across the phase transition. These quantities include the spin polarization, the relative occupation of the nearly degenerate single-particle states, the quantity analogous to the photon field occupation and the period of a collective oscillation (quadrupole mode). The applicability of the Dicke model to spin-orbit-coupled BECs may lead to interesting applications in quantum optics and quantum information science. Ultracold atomic gases afford unique opportunities to simulate quantum optical and condensed matter phenomena, many of which are difficult to observe in their original contexts [1] , [2] . Over the past decade, much theoretical and experimental progress in implementing quantum simulations with atomic gases has been achieved, exploiting the flexibility and tunability of these systems. The recent generation of spin-orbit (SO) coupling in Bose–Einstein condensates (BECs) [3] , [4] , [5] , [6] and Fermi gases [7] , [8] , [9] has brought the simulation of a large class of gauge field-related physics into reach, such as the spin Hall effect [10] , [11] , [12] , [13] . With such achievements, SO-coupled ultracold atomic gases have emerged as excellent platforms to simulate topological insulators, topological superconductors/superfluids and so on, which have important applications for the design of next-generation spin-based atomtronic devices and for topological quantum computation [14] , [15] . Recently, the ground state properties of a BEC with one-dimensional (1D) or two-dimensional (2D) SO coupling have been analysed theoretically. These investigations have predicted a plane wave or stripe phase for different parameter regimes [16] , [17] , [18] , [19] , [20] , [21] , [22] , [23] , agreeing with the experimental observations [3] . In the plane wave phase of such a SO-coupled BEC, the atomic spins collectively interact with the motional degrees of freedom in the external trapping field, providing a possible analogy to the well-known quantum Dicke model. The Dicke model [24] , proposed nearly 60 years ago, describes the interaction between an ensemble of two-level atoms and an optical field [25] . For atom–photon interaction strengths greater than a threshold value, the ensemble of atoms favours to interact with the optical field collectively as a large spin and the system shows an interesting superradiant phase with a macroscopic occupation of photons and non-vanishing spin polarization [26] , [27] , [28] . Even though this model has been solved and is well understood theoretically, the experimental observation was achieved only recently by coupling a BEC to an optical cavity [29] . In this work, we experimentally investigate the ground state properties of the plane wave phase of a SO-coupled BEC and show that an insightful analogy to the quantum optical Dicke model can be constructed. The SO coupling in a BEC is realized with a Raman dressing scheme. The system exhibits coupling between momentum states and the collective atomic spin, which is analogous to the coupling between the photon field and the atomic spin in the Dicke model. This analogy is depicted in Fig. 1 . By changing the Raman coupling strength, the system can be driven across a quantum phase transition from a spin-polarized phase, marked by a non-zero quasi-momentum, to a spin-balanced phase with zero quasi-momentum, akin to the transition from superradiant to normal phases in Dicke model. Measurements of various physical quantities in these two phases are presented. 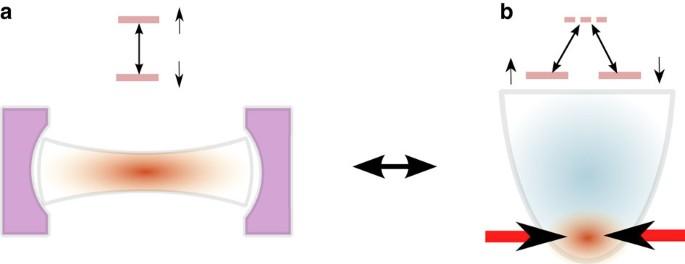Figure 1: Analogy between standard Dicke model and SO-coupled BEC. (a) Standard Dicke model describing the interaction of an ensemble of two-level atoms in an optical cavity. The optical mode in the cavity couples two atomic spin states. (b) SO-coupled BEC in an external trap. Two spins states are coupled by two counter-propagating Raman lasers. Figure 1: Analogy between standard Dicke model and SO-coupled BEC. ( a ) Standard Dicke model describing the interaction of an ensemble of two-level atoms in an optical cavity. The optical mode in the cavity couples two atomic spin states. ( b ) SO-coupled BEC in an external trap. Two spins states are coupled by two counter-propagating Raman lasers. Full size image Theoretical description of the SO-coupled BEC The Raman dressing scheme is based on coupling two atomic hyperfine states in such a way that a momentum transfer of 2 ℏ k R in the x direction is accompanied with the change of the hyperfine states, where ℏ k R is the photon recoil momentum. The dynamics in the y and z directions are decoupled, which allows us to consider a 1D system in our following discussions (see Methods). The two coupled hyperfine states are regarded as the two orientations of a pseudo-spin 1/2 system. The Raman dressed BEC is governed by the 1D Gross–Pitaevskii (G-P) equation with the Hamiltonian H SO = H s + H I . Here H s is the single-particle Hamiltonian and in the basis of the uncoupled states can be written as Ω is the Raman coupling strength and δ is the detuning of the Raman drive from the level splitting. The recoil energy is defined as E R = ℏ 2 k R 2 /2 m . k x is the quasi-momentum and V t = mω x 2 x 2 /2 is the external harmonic trap. The many-body interactions between atoms are described by where g αβ are the effective 1D interaction parameters (see Methods) [30] , [31] . The presence of the interatomic interactions is crucial to observe the Dicke phase transition. For 87 Rb atoms, the differences between the spin-dependent nonlinear coefficients are very small and contribute only small modifications to the collective behaviour (see Methods). The band structure of the non-interacting system with Ω<4 E R and δ =0 has two degenerate local minima at quasi-momenta ± q , where q = k R (1−(Ω/4 E R ) 2 ) 1/2 . The spin polarization of these two states is finite and opposite to each other. An ensemble of non-interacting atoms occupies both states equally and thus has zero average spin polarization and quasi-momentum. When the nonlinear interactions are taken into account, a superposition state with components located at both degenerate minima generally has an increased energy and is thus not the many-body ground state [32] . The ground state of the BEC is obtained when the atoms occupy one of the degenerate single-particle ground states (L or R). This is depicted in the inset of Fig. 2a . 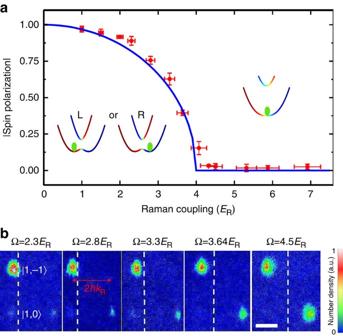Figure 2: Spin polarization and corresponding quasi-momentum from time-of-flight image. (a) Absolute value of the spin polarization as a function of Raman coupling strength Ω forδ=0. The solid blue line gives the spin polarization predicted by the Dicke model. The symbols are the experimentally measured data. The vertical error bars are the s.d. for 4–5 realizations, while the horizontal error bars reflect the systematic uncertainties in the determination of Ω. The insets are examples of the dispersion relation in the regime of Ω below or above 4ER, and the colour of the bands represents the spin composition. (b) Example of experimental time-of-flight images of BECs loaded to +q. The pseudo-spin states are horizontally separated by 2ℏkRdue to the Raman momentum transfer and the dashed vertical line indicates zero momentum. The separation of the spin states in the vertical direction is achieved by a Stern–Gerlach field which is briefly applied during time-of-flight. The inset scale bar corresponds to 50 μm. Figure 2: Spin polarization and corresponding quasi-momentum from time-of-flight image. ( a ) Absolute value of the spin polarization as a function of Raman coupling strength Ω for δ =0. The solid blue line gives the spin polarization predicted by the Dicke model. The symbols are the experimentally measured data. The vertical error bars are the s.d. for 4–5 realizations, while the horizontal error bars reflect the systematic uncertainties in the determination of Ω. The insets are examples of the dispersion relation in the regime of Ω below or above 4 E R , and the colour of the bands represents the spin composition. ( b ) Example of experimental time-of-flight images of BECs loaded to + q . The pseudo-spin states are horizontally separated by 2 ℏ k R due to the Raman momentum transfer and the dashed vertical line indicates zero momentum. The separation of the spin states in the vertical direction is achieved by a Stern–Gerlach field which is briefly applied during time-of-flight. The inset scale bar corresponds to 50 μm. Full size image The mean field energy associated with a spin-flip in an interacting, harmonically trapped BEC is determined by the coupling between the atomic spin and the many-body ground state harmonic mode. This situation is similar to that of many two-level atoms interacting with a single photon field in an optical cavity [24] . As shown in the following, the interaction-induced spontaneous symmetry breaking of the ground state allows the mapping of the SO-coupled BEC to the well-known Dicke model, leading to the prediction of an intriguing quantum phase transition when the Raman coupling strength is varied [33] . Mapping to the Dicke model The realization of the Dicke transition requires two conditions: a single mode that interacts with all atoms and the thermodynamic (large atom number) limit. While the latter is naturally fulfilled in our SO-coupled BECs with N >10 4 atoms, the first condition is driven by the many-body interaction between atoms. Note that the mean field interaction energy contains two types of terms (see Methods): a term proportional to the overall interaction strength ( ∝ g ↑↑ + g ↓↓ +2 g ↑↓ ) that prefers a uniform density (the plane wave phase) and a term proportional to the difference of the interaction strengths in different spin states ( ∝ g ↑↑ −g ↑↓ ) that prefers spatial modulation of the density. In the experiment, the first term dominates for a reasonably large Ω and the plane wave phase is preferred (that is, possesses the lowest energy) [22] . In this phase, all atoms collectively interact with a single plane wave mode, similar to atoms confined in a cavity interacting only with the cavity mode. To see the connection between the SO-coupled BEC and the Dicke model, the interacting many-body ground state is first expressed in terms of the harmonic trap mode (see Methods). Setting p x = ℏ k x = i ( mω x ℏ /2) 1/2 ( a † − a ), the N -particle Hamiltonian can be written as where the uniform approximation has been adopted to treat the nonlinear interaction term, , n is the local density. J x , z are the collective spin operators defined as is the occupation number of the harmonic trap mode. The differences between the interaction energies contribute an effective detuning term and a nonlinear term in the large spin operator, . However, these terms are small for the experimental states chosen and thus are ignored in the following analysis. For δ =0, the Hamiltonian of the first line in equation (3) is equivalent to the Dicke model [24] . A quantum phase transition between the normal phase and a superradiant phase can be driven by changing the Raman coupling strength Ω. The critical point for the phase transition can be derived using the standard mean field approximation [34] , [35] , [36] yielding Ω c =4 E R (note that the term yields a small correction −4 G 3 / N to Ω c , which is neglected here). When Ω<Ω c , the Dicke model predicts that the dependence of the order parameter on the Raman coupling strength is . For Ω>Ω c , one obtains 〈 J z 〉/ j ℏ =0 and 〈 σ x 〉=〈 J x 〉/ j ℏ =1 ( j = N /2). This scaling is confirmed in our numerical simulation of the G-P equation. The ground state of the BEC is obtained through an imaginary time evolution. The spin polarization can be calculated as . The absolute value of 〈 σ z 〉 is taken since ± q are spontaneously chosen. The scaling of |〈 J z 〉|/( j ℏ ) is shown in Fig. 2 and clearly is consistent with the experimental data described in the following. Experimental procedure To experimentally probe this system, we adiabatically Raman dress a BEC of 87 Rb atoms in the and hyperfine states (see Methods). A magnetic bias field is applied that generates a sufficiently large quadratic Zeeman splitting such that the | F =1, m F =1〉 state can be neglected. The system can thus be treated as an effective two-state system. To analyse the bare state composition, all lasers are switched off and the atoms are imaged after time-of-flight in a Stern–Gerlach field. This separates the bare states along the vertical axis of the images. The absolute value of the spin polarization, given by |( N ↑ – N ↓ )|/( N ↑ + N ↓ ), and the quasi-momentum are directly measured for condensed atoms at ± q . The experimentally measured absolute value of the spin polarization for various Raman coupling strengths Ω spanning the quantum phase transition is shown in Fig. 2a . An experimental investigation of the collective choice of the atoms to occupy a single minimum in the dispersion relation is presented in Fig. 3 . For this data, the BEC is adiabatically prepared in a Raman dressed state with Ω=3 E R and a detuning δ of either ±5.4 E R . The detuning is then linearly swept to a final value in 50 ms. The left/right relative occupation of the BEC, defined by ( N + q – N − q )/( N + q + N − q ), provides a measure for the relative occupation of the dressed states at the quasi-momentum of the two dispersion minima. The data presented in Fig. 3 exhibits a hysteretic effect dependent on the sign of the initial detuning ± δ . The width of the hysteresis depends on the chosen sweep rate of the detuning (see Methods). While these sweeps are slow enough for the BEC to follow a chosen minimum of the band structure, the transition between the two possible minima is non-adiabatic. Sweeps causing a reversal of the energetic order of the two minima eventually generate heating of the BEC, shown in Fig. 3c . Only values of δ where the BEC is not heated are plotted in Fig. 3a,b . Recently, a similar energy dispersion exhibiting a double well structure was also observed for a BEC in a shaken optical lattice, where the analogous spontaneous occupation of a single band mimimum was also found [37] . However, such a system lacks the linear coupling between momentum and spin presented in our system (Equation 1), and thus cannot be mapped to the Dicke model. 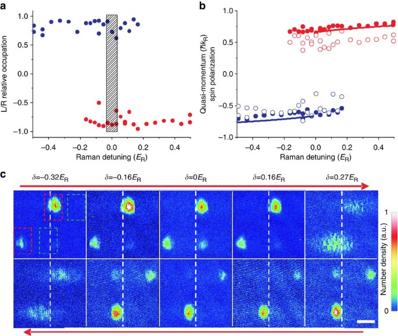Figure 3: Effect of a small detuning on the superradiant phase. (a) Experimentally measured relative occupation of the two dispersion minima in the superradiant phase. The system is loaded adiabatically for Ω=3ERat a detuning of −5.4ER(blue points) or +5.4ER(red points). Then the detuning is linearly swept to the final value in 50 ms. The hashed region indicates the experimental uncertainty to whichδ=0 is determined. (b) Experimental measurements of the spin polarization (open circles) and quasi-momentum (filled circles) overlaid with the single-particle expectations (lines). (c) Absorption images taken after projecting the BEC onto the bare states, applying Stern–Gerlach separation and 11.5 ms time of flight. The given values ofδare the endpoints of the detuning ramps described in the main text. The relative occupation inais calculated from the atom numbers contained in the dashed boxes inc. The dashed vertical line indicates zero kinetic momentum, while the horizontal red arrows indicate the direction in whichδis swept. The inset scale bar is 50 μm. Figure 3: Effect of a small detuning on the superradiant phase. ( a ) Experimentally measured relative occupation of the two dispersion minima in the superradiant phase. The system is loaded adiabatically for Ω=3 E R at a detuning of −5.4 E R (blue points) or +5.4 E R (red points). Then the detuning is linearly swept to the final value in 50 ms. The hashed region indicates the experimental uncertainty to which δ =0 is determined. ( b ) Experimental measurements of the spin polarization (open circles) and quasi-momentum (filled circles) overlaid with the single-particle expectations (lines). ( c ) Absorption images taken after projecting the BEC onto the bare states, applying Stern–Gerlach separation and 11.5 ms time of flight. The given values of δ are the endpoints of the detuning ramps described in the main text. The relative occupation in a is calculated from the atom numbers contained in the dashed boxes in c . The dashed vertical line indicates zero kinetic momentum, while the horizontal red arrows indicate the direction in which δ is swept. The inset scale bar is 50 μm. Full size image From the effective Dicke model, we also obtain the quantity analogous to the photon field excitation, as well as the ground state energy of the system. The photon number N p is related to the quasi-momentum q of the SO-coupled BEC: N p = q 2 after a constant coefficient is scaled to unity (see Methods). As seen from the experimental measurements and numerical simulations in Fig. 4a , the superradiant phase has a macroscopic photon excitation, while the photon field vanishes in the normal phase. The ground state energy E s of a single particle, as obtained from G-P simulations, is plotted in Fig. 4b and is in agreement with the predictions of the Dicke model. The second-order derivative of E s is discontinuous at the critical point Ω=4 E R , reinforcing the nature of the quantum phase transition. The red circles in Fig. 4b show the density-dependent mean field interaction energy in the numerical simulations, contributing ~0.2 E R to the total energy. 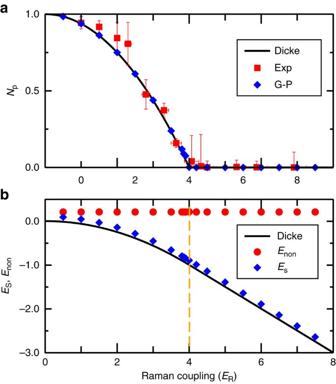Figure 4: Photon field excitation and ground state energy. (a) Scaled photon field excitation of the effective Dicke model. The red symbols are the experimental results from the quasi-momentum measurements. The vertical error bars are the s.d. for 4–5 realizations, while the horizontal error bars reflect the systematic uncertainties in the determination of Ω. The blue symbols are the simulation results based on the G-P equation and the solid line is the prediction of the Dicke model. (b) Numerical results for the single-particle ground state energyEs(blue diamonds) and the nonlinear interaction energyEnon(red circles) as a function of Raman coupling strength. The black solid line shows the single-particle energy from the prediction of the Dicke model. The dashed vertical line indicates the location of the quantum phase transition. Figure 4: Photon field excitation and ground state energy. ( a ) Scaled photon field excitation of the effective Dicke model. The red symbols are the experimental results from the quasi-momentum measurements. The vertical error bars are the s.d. for 4–5 realizations, while the horizontal error bars reflect the systematic uncertainties in the determination of Ω. The blue symbols are the simulation results based on the G-P equation and the solid line is the prediction of the Dicke model. ( b ) Numerical results for the single-particle ground state energy E s (blue diamonds) and the nonlinear interaction energy E non (red circles) as a function of Raman coupling strength. The black solid line shows the single-particle energy from the prediction of the Dicke model. The dashed vertical line indicates the location of the quantum phase transition. Full size image Collective excitations It is well known that various physical quantities may change dramatically across a quantum critical point [38] . As a particular example, we investigate the quadrupole collective excitation of a SO-coupled BEC. In BECs without SO coupling, the quadrupole excitation frequency only depends on the trapping geometry and on the ratio of the kinetic energy to the trapping energy [39] . Measurements and G-P simulations of the quadrupole-mode frequencies for SO-coupled BECs are shown in Fig. 5 as a function of the Raman coupling strength. For this data, the quadrupole oscillation period is scaled by the period measured for an off-resonant case . This removes a dependence on the trapping geometry that changes with the Raman coupling strength in the experiment. A peak in the oscillation period around the phase transition is observed. In the G-P simulations, a quadrupole oscillation amplitude of ~0.2 ℏ k R was used, whereas the oscillation amplitude in the experimental results varied from 0.15 ℏ k R to 0.55 ℏ k R . In SO-coupled systems, the hydrodynamic-mode frequencies depend strongly on the oscillation amplitude [4] . This may contribute to the variation of the experimental data. The numerical results reveal that the oscillations of the BEC are undamped in both spin-balanced and -polarized phases, but show strong damping in the transition region. The behaviour of the quadrupole mode provides an additional signature of the quantum phase transition. Similar experimental behaviour has been observed for the collective dipole motion [4] . 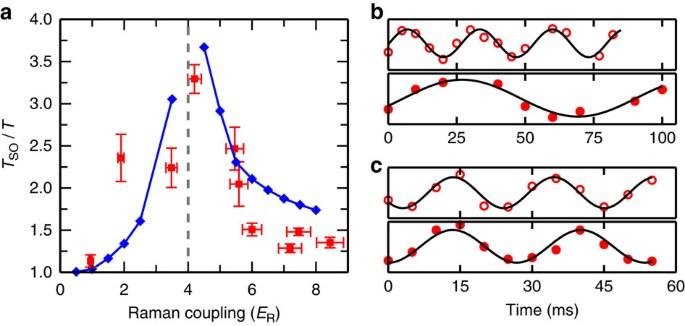Figure 5: Quadrupole excitations across the Dicke phase transition. (a) Scaled quadrupole oscillation period forδ≈0. The blue points and the solid blue line are the results of numerical simulations. The dashed vertical line indicates the location of the quantum phase transition. The red symbols with error bars are the experimentally measured data. The vertical error bars are the uncertainty of the oscillation frequency from the sinusoidal fits, while the horizontal error bars reflect the systematic uncertainties in the determination of Ω. (b,c) Experimentally observed temporal oscillation of the condensate width for (b) Ω=4.2ERand (c) Ω=7.2ER. The upper and lower panels of each figure represent the off-resonant case () and on-resonant case (δ≈0), respectively. The solid lines are fits to the experimental data. Figure 5: Quadrupole excitations across the Dicke phase transition. ( a ) Scaled quadrupole oscillation period for δ ≈0. The blue points and the solid blue line are the results of numerical simulations. The dashed vertical line indicates the location of the quantum phase transition. The red symbols with error bars are the experimentally measured data. The vertical error bars are the uncertainty of the oscillation frequency from the sinusoidal fits, while the horizontal error bars reflect the systematic uncertainties in the determination of Ω. ( b , c ) Experimentally observed temporal oscillation of the condensate width for ( b ) Ω=4.2 E R and ( c ) Ω=7.2 E R . The upper and lower panels of each figure represent the off-resonant case ( ) and on-resonant case ( δ ≈0), respectively. The solid lines are fits to the experimental data. Full size image Finite detuning While the analysis above has focused on the case of δ =0, a finite detuning leads to the realization of the generalized Dicke Hamiltonian [40] . For finite detuning, the sharp quantum phase transition vanishes and the BEC is always in a superradiant (spin-polarized) phase, as shown in Fig. 6 . The inclusion of this parameter demonstrates the completeness in the mapping of the SO-coupled BEC to a Dicke-type system. 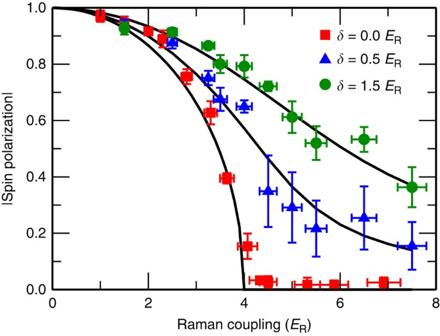Figure 6: Realization of a generalized Dicke model. Absolute value of the spin polarization as a function of Raman coupling strength Ω for detuningsδ=0ER, 0.5ERand 1.5ER. For a finite detuning there is only one non-degenerate solution of the generalized Dicke model and no quantum phase transition exists. The data points are experimental measurements and the solid lines are the corresponding theoretical predictions from the generalized Dicke model. The vertical error bars are the s.d. for 4–5 realizations, while the horizontal error bars reflect the systematic uncertainties in the determination of Ω. Figure 6: Realization of a generalized Dicke model. Absolute value of the spin polarization as a function of Raman coupling strength Ω for detunings δ =0 E R , 0.5 E R and 1.5 E R . For a finite detuning there is only one non-degenerate solution of the generalized Dicke model and no quantum phase transition exists. The data points are experimental measurements and the solid lines are the corresponding theoretical predictions from the generalized Dicke model. The vertical error bars are the s.d. for 4–5 realizations, while the horizontal error bars reflect the systematic uncertainties in the determination of Ω. Full size image We have demonstrated that varying the Raman coupling strength can drive a harmonically trapped SO-coupled BEC across a quantum phase transition from a spin-balanced to a spin-polarized ground state. This is a realization of the long-sought phase transition from a normal to a superradiant phase in the quantum Dicke model. The corresponding spin polarization and photon field occupation are calculated for the Dicke model and agree with the experimental measurements and the numerical simulations. The ground state energy is found to be consistent with our numerical simulations as well. Using SO-coupled BECs to study the Dicke model physics may have important applications in quantum information and quantum optics including spin squeezing, quantum entanglement and so on. Experimental set-up and parameters For the experiments presented in this article, the BECs are held in a crossed optical dipole trap with frequencies { ω x , ω y , ω z ,} within the range of 2π × {12–34,134,178} Hz, respectively. Depending on the Raman coupling strength and crossed dipole trap potential, BECs of 2 × 10 4 to 10 × 10 4 atoms are loaded into the dressed state. Small atom numbers are favourable in this trapping geometry to reduce collisions between atoms differing by 2 ℏ k R during time-of-flight. The Raman beams, intersecting under an angle of π/2, are individually oriented at an angle of π/4 from the long axis of the BEC. They are operated between the D1 and D2 lines of 87 Rb in the range of 782.5−790 nm. A 10-G magnetic bias field is applied along the long axis of the BEC and produces a quadratic Zeeman shift of ~7.4 E R . The BEC is imaged after performing Stern–Gerlach separation during a 11.5-ms time-of-flight expansion. The images directly reveal the spin and momentum distributions. For each value of Ω, δ =0 is experimentally identified by finding the Raman laser detuning for which the spin polarization is minimized (normal phase) or for which the BEC switches between the two degenerate states (superradiant phase). This method compensates for the presence of the third atomic hyperfine state (|1, +1〉) in the F =1 manifold. The magnetic bias field was actively stabilized using a technique similar to the one described in ref. 41 . Experimental preparation methods To experimentally measure the absolute value of the spin polarization |〈 σ z 〉| and the photon field occupation (shown in Figs 2 and 4 ), we start with a BEC in the bare state and adiabatically turn on the Raman dressing at δ =5.4 E R (−5.4 E R ). The initial state and the dressed state have similar spin compositions. This is followed by a linear sweep of the detuning to a final value in 50–100 ms. An example of results obtained with this loading method is shown in Fig. 7 for the normal phase of the Dicke model with Ω=6 E R . This loading method produces BECs with only minimal excitations when the final detuning value is chosen near δ =0. As seen in Fig. 3 , this method can cause a hysteresis-like feature at small | δ |. 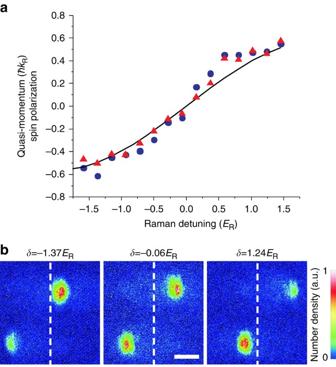Figure 7: Effect of a small detuning on the normal phase. (a) Spin polarization (triangles) and quasi-momentum (circles) measured for the normal phase, where there is no degeneracy in the ground state of the single-particle dispersion. This measurement was performed at Ω=6ERfor variousδ. The data are overlaid with the single-particle expectation for the ground state of the system (solid line). (b) Experimental images for three different realizations ina. The dashed vertical line indicates zero momentum. The inset scale bar corresponds to 50 μm. Figure 7: Effect of a small detuning on the normal phase. ( a ) Spin polarization (triangles) and quasi-momentum (circles) measured for the normal phase, where there is no degeneracy in the ground state of the single-particle dispersion. This measurement was performed at Ω=6 E R for various δ . The data are overlaid with the single-particle expectation for the ground state of the system (solid line). ( b ) Experimental images for three different realizations in a . The dashed vertical line indicates zero momentum. The inset scale bar corresponds to 50 μm. Full size image An alternative loading method, as opposed to ramps of δ , is investigated by fixing the laser detuning while Ω is increased. The resulting L/R relative occupation measurement is shown in Fig. 8 . Here the BEC is loaded to the desired parameters in ~60 ms by only increasing the Raman beam intensities. This is followed by a 150-ms wait time, allowing for excitations to be dissipated. While this wait time is long, there may still be some residual small amplitude collective excitations, such as dipole oscillations. When this technique is used in Fig. 8 , the BEC occupies only one of the two minima for all but small detunings. In the range where the BEC fails to load to a single point in the dispersion relation, the quasi-momentum (shown in Fig. 8b , strongly deviates from the single-particle expectation and the BEC acquires excitations. While this loading method does not result in the occupation of the ground state at δ =0, the BEC does choose a single minimum for detunings much smaller than the chemical potential μ , which is on the order of 0.55 E R for the data shown. Similar results are obtained by adding sufficient wait time following the linear sweeps of δ performed for Fig. 3 . A related effect has been observed in ref. 42 . 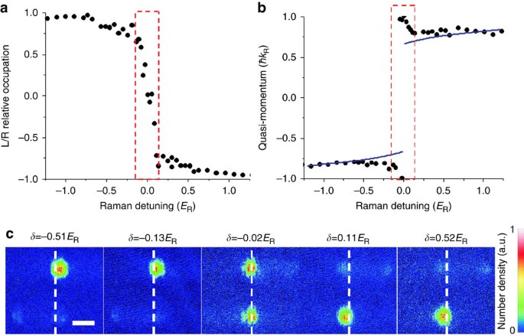Figure 8: Effect of a small detuning on the superradiant phase using an alternative loading method. (a) Experimental determination of the L/R relative occupation of the BEC in the superradiant phase for Ω=3ER. The Raman coupling is ramped on over 60 ms at a fixed laser detuning (which differs from the condition of fixedδ) followed by a 150-ms wait time. For all but small detunings the system is loaded to a single point in the dispersion relation. (b) The accompanying quasi-momentum deviates from the expected single-particle value (solid lines) at small detunings where the BEC acquires excitations. This region is highlighted by the dashed red boxes. (c) Experimental images. The inset scale bar corresponds to 50 μm. Figure 8: Effect of a small detuning on the superradiant phase using an alternative loading method. ( a ) Experimental determination of the L/R relative occupation of the BEC in the superradiant phase for Ω=3 E R . The Raman coupling is ramped on over 60 ms at a fixed laser detuning (which differs from the condition of fixed δ ) followed by a 150-ms wait time. For all but small detunings the system is loaded to a single point in the dispersion relation. ( b ) The accompanying quasi-momentum deviates from the expected single-particle value (solid lines) at small detunings where the BEC acquires excitations. This region is highlighted by the dashed red boxes. ( c ) Experimental images. The inset scale bar corresponds to 50 μm. Full size image The quadrupole frequency measurements begin with a BEC in the | F , m F 〉=|1, −1〉 state in the crossed dipole trap. The two Raman beam intensities are linearly increased, one after the other, over 30–150 ms. This loading method, performed with the Raman beams at 782.5 nm, generates large quadrupole and small dipole excitations. To simplify the analysis, only the first few oscillations of the quadrupole mode are fit to an undamped oscillation. In the numerical simulations, the quadrupole mode is excited by a sudden jump of the trap frequency along the SO coupling direction. Evolution time is added to observe the temporal oscillation of the condensate width that reveals the quadrupole-mode frequency. Dimension reduction from 3D to 1D The dynamics of SO-coupled BECs and their mapping to the Dicke model are studied on the basis of the 1D G-P equation, although the experimental system is three dimensional (3D) with strong confinements along two directions. The SO coupling is along the elongated direction of the trap, therefore the transverse degrees of freedom do not couple with the internal spin states. Assuming the harmonic ground states along the transverse directions, the effective 1D nonlinear interaction coefficients, g 1D , can be approximately obtained from 3D through g 1D = g 3D / l y l z , where are the harmonic characteristic lengths along the transverse directions and is the 3D nonlinear interaction coefficient. For the study of the quadrupole mode, we simulate the 2D G-P equation in the xy plane to compare with the experimental observations, where the dimension reduction gives g 2D = g 3D / l z . Mapping to the Dicke-type Hamiltonian In the mean field approximation, the single-particle Hamiltonian is given by As discussed in the main text, the large nonlinear interactions enable the atoms to collectively occupy the same many-body ground state, forming a single mode. For an ensemble of N interacting bosonic atoms, we define the collective spin operators and . Substituting these collective operators into the N -particle Hamiltonian and using the harmonic mode operator, , we obtain which corresponds to the generalized Dicke model. The interaction term in the mean field approximation is which can also be formally expressed using collective operators. We define the variables , and (ref. 22 ), where n is the average density of the BEC. For the parameters used in our experiment, we have , thus G 3 =2 G 2 ≈0 and . Because of the normalization condition of the BEC wave function, it is easy to see that and ( J z = N ℏ /2 when all atoms are in the spin-up state). With these notations, the Hamiltonian can be mapped to Note that is proportional to N , thus all the terms in the above Hamiltonian scale as N . Dicke phase transition The critical point for the phase transition of the Dicke model can be derived using the mean field coherent state [36] , where the mean field ansatz of the ground state wave function is given by Here the spatial coherent state | α 〉 is defined by a | α 〉= α | a 〉, and the spin coherent state | θ 〉 is defined as with j = N /2 for spin 1/2 atoms and θ ∈ [0,2 π ]. In the absence of the detuning term , the ground state energy of the Dicke Hamiltonian is where u and v are the real and imaginary parts of α , that is, α = u + iv . Minimizing E ( θ , α ) with respect to u and v leads to Thus the ground state energy becomes Further minimization of E ( θ , α ) with respect to θ leads to Defining Ω c =4 E R (1−G 3 / NE R ), we obtain two different regions: 1 Ω>Ω c : there is only one solution that minimizes the mean field energy: cos θ =0 and sin θ =−1. In this case, the spin polarization is zero and the corresponding phase is the spin-balanced normal phase. 2 Ω<Ω c : the energy is minimized for and there are two possible values for , corresponding to a BEC occupying the left or right band minimum. Ground state properties in the Dicke model In the following, we neglect the constant mean field energy terms and the small G 3 terms, therefore Ω c ≈4 E R . In the region Ω>Ω c , the system is in the normal phase and v = u =0. The mean photon number is The spin polarizations become The ground state energy per particle is We denote the first two terms as the single-particle energy E s . In the region Ω<Ω c , the system is in the superradiant phase with and the mean photon number where is the quasi-momentum of the BEC. Note that the average photon number depends on the trapping frequency and in the main text we rescale it to . The spin polarization in the superradiant phase is Finally, the ground state energy per particle is We denote the first term as the single-particle energy E s . The energy expressions for Ω<4 E R and Ω>4 E R are consistent, they are continuous at Ω=4 E R . How to cite this article: Hamner, C. et al. Dicke-type phase transition in a spin-orbit coupled Bose-Einstein condensate. Nat. Commun. 5:4023 doi: 10.1038/ncomms5023 (2014).